Targeting cell surface TLR7 for therapeutic intervention in autoimmune diseases Toll-like receptor 7 (TLR7) senses microbial-derived RNA but can also potentially respond to self-derived RNA. To prevent autoimmune responses, TLR7 is thought to localize in endolysosomes. Contrary to this view, we show here that TLR7 is present on the cell surface of immune cells and that TLR7 responses can be inhibited by an anti-TLR7 antibody. The anti-TLR7 antibody is internalized with TLR7 and accumulates in endolysosomes as an immune complex. TLR7 responses in dendritic cells, macrophages and B cells are all inhibited by the anti-TLR7 antibody. Furthermore, the anti-TLR7 antibody inhibits in vivo cytokine production induced by a TLR7 ligand. Spontaneous TLR7 activation in Unc93b1 D34A/D34A mice causes lethal inflammation. Progressive inflammation such as splenomegaly, thrombocytopenia and chronic active hepatitis are ameliorated by anti-TLR7 antibody treatment. These results demonstrate that cell surface TLR7 is a promising target for therapeutic intervention in autoimmune diseases. Toll-like receptors (TLRs) sense a variety of microbial products such as microbial membrane lipids or nucleic acids (NAs) and initiate innate and adaptive immune responses [1] , [2] . Toll-like receptors 7 (TLR7) and 9 (TLR9), which act as innate immune sensors of microbial NAs [3] , erroneously respond to self-NAs, thus inducing antinuclear autoantibody production in murine models of systemic lupus erythematosus (SLE) [4] , [5] , [6] . Self-pathogen discrimination by TLR7 or TLR9 is error-prone, and the restriction of NA sensing in endolysosomes is believed to prevent autoimmunity [7] . Whereas self-derived NAs are rapidly degraded by nucleases, microbial NAs are resistant to degradation because they are encased in bacterial cell walls or viral particles. Microbial NAs are therefore able to reach endolysosomes to stimulate TLR7 or TLR9 (ref. 8 ). The aberrant transportation of self-NAs to endolysosomes has been shown to exacerbate autoimmunity [6] , [9] , [10] . In addition to ligand transportation, sensor transportation is also tightly controlled to prevent autoimmunity. If TLR9 is forced to be expressed on the cell surface, TLR9 signals in response to extracellular self DNA lead to systemic lethal inflammation [11] . The trafficking of TLR7 and TLR9 out of the endoplasmic reticulum (ER) is dependent on Unc93B1, a multiple transmembrane protein associated with TLR7 or TLR9 (refs 12 , 13 ). Unc93B1 also plays a role in balancing between TLR7 and TLR9 responses. A point mutation of aspartic acid at position 34 (D34A) alters the balance of TLR7 and TLR9 toward TLR7 (refs 14 , 15 ), leading to TLR7-dependent systemic lethal inflammation. In lupus-prone mouse strains such as MRL/lpr and C57BL/6 mice congenic for Nba2 (New Zealand Black autoimmunity 2), TLR7 exacerbates lupus nephritis, whereas TLR9 regulates disease progression by counteracting TLR7 (refs 4 , 14 , 16 , 17 ). Thus, TLR7-dependent signalling is likely to promote autoimmune diseases. Oligodeoxynucleotides that antagonize TLR7, 8 and 9 ameliorate disease conditions in psoriasis and SLE mouse models [18] , [19] , demonstrating that NA-sensing TLRs, are promising targets in treating psoriasis or SLE. Although antibodies (Abs) are powerful tools for therapeutic intervention, TLR7 has been excluded from the list of targets for Ab-mediated intervention because of its lack of cell surface expression. Despite this expectation, we found that an anti-TLR7 Ab inhibits TLR7 responses both in vitro and in vivo . Moreover, TLR7-dependent inflammation in Unc93b1 D34A/D34A mice was ameliorated by anti-TLR7 Ab treatment. The anti-TLR7 Ab targets TLR7 on the cell surface of immune cells and is internalized to endolysosomes. These results demonstrate that cell surface TLR7 is an unexpected and promising target for therapeutic intervention in autoimmune diseases. Unc93B1-dependent expression of TLR7 on the cell surface TLR7 is believed to reside in intracellular vesicles to prevent autoimmune responses to self RNA. A recently characterized anti-mouse TLR7 monoclonal Ab (mAb) [20] was used to reveal cell surface TLR7 on bone marrow-derived macrophages (BM-MCs; Fig. 1a ). The specificity was verified by staining Tlr7 −/− BM-MCs. Cell surface TLR7 expression on BM-conventional dendritic cells (BM-cDCs), BM-plasmacytoid DCs (BM-pDCs) and B cells was much lower than that on BM-MCs but was still detectable. Membrane-permeabilized staining showed that the cell surface expression of TLR7 did not necessarily correlate with the total amount of TLR7. Although BM-pDCs expressed TLR7 as highly as BM-MCs, the cell surface TLR7 on BM-pDCs was much lower than that on BM-MCs, suggesting the existence of a mechanism specifically controlling cell surface TLR7 expression. To confirm cell surface TLR7 expression in vivo , splenic DCs were stained. TLR7 was appreciably detected on splenic pDCs and all of the cDC subsets ( Fig. 1b ). Unc93B1, a multiple transmembrane protein, associates with TLR7 or 9 and transports them from the ER to endolysosomes [13] , [15] , [21] . Our recent study shows that TLR9 is expressed on the surface of splenic DCs in a Unc93B1-dependent manner [21] . Cell surface TLR7 expression was also dependent on Unc93B1 because cell surface TLR7 was not detected on splenic DCs from Unc93b1 3d/3d mice, which harbour a loss-of-function mutation in the Unc93b1 gene ( Fig. 1b ) [12] . Cell surface TLR7 was also detected on macrophage cell lines and peripheral blood monocytes ( Supplementary Fig. 1 ). These results demonstrate that TLR7 is expressed on the surface of innate immune cells. 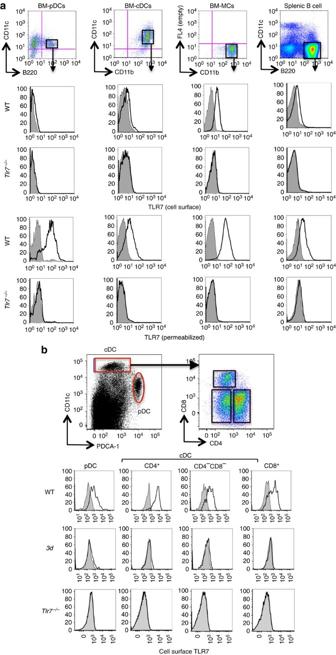Figure 1: TLR7 is expressed on the cell surface. (a) Dot plots show the maturation status of BM-pDCs, BM-cDCs, BM-MCs and splenic B cells from wild-type (WT) mice using the indicated surface markers. Open histograms show cell surface (upper) and membrane-permeabilized (lower) staining with the anti-TLR7 mAb. Shaded histograms show staining with the secondary reagent alone. Cells fromTlr7−/−mice are shown as negative controls. (b) Dot plots show the FACS profiles of splenic cells from WT mice. CD11chiPDCA-1locDCs were further subdivided into three subsets by the expression of CD4 and CD8. Open histograms show cell surface TLR7 on DC subsets, and shaded histograms represent negative controls stained with the secondary reagent alone. The results usingUnc93b13d/3d(3d) andTlr7−/−mice are also shown. These data are representative of three independent experiments. Figure 1: TLR7 is expressed on the cell surface. ( a ) Dot plots show the maturation status of BM-pDCs, BM-cDCs, BM-MCs and splenic B cells from wild-type (WT) mice using the indicated surface markers. Open histograms show cell surface (upper) and membrane-permeabilized (lower) staining with the anti-TLR7 mAb. Shaded histograms show staining with the secondary reagent alone. Cells from Tlr7 −/− mice are shown as negative controls. ( b ) Dot plots show the FACS profiles of splenic cells from WT mice. CD11c hi PDCA-1 lo cDCs were further subdivided into three subsets by the expression of CD4 and CD8. Open histograms show cell surface TLR7 on DC subsets, and shaded histograms represent negative controls stained with the secondary reagent alone. The results using Unc93b1 3d/3d ( 3d ) and Tlr7 −/− mice are also shown. These data are representative of three independent experiments. Full size image Anti-TLR7 mAb inhibits TLR7 responses in vitro To study the effect of the mAb on TLR7 responses, anti-TLR7 mAb was added in vitro to cells before stimulation by a variety of TLR7 ligands. Although TLR7 is thought to be activated in endolysosomes, exogenously added anti-TLR7 mAb completely inhibited the production of cytokines, including interleukin (IL)-6, tumour necrosis factor (TNF )-α and RANTES (CCL5), by BM-MCs stimulated with TLR7 ligands such as the base analogue loxoribine and the synthetic RNA RNA9.2 (ref. 22 ; Fig. 2a and Supplementary Fig. 2a ). Cytokine production by the TLR9 ligand CpG-B was not altered. TLR7-specific inhibition was also observed in BM-cDCs and BM-pDCs ( Fig. 2b,c ), although both types of cells showed very low TLR7 expression on the cell surface ( Fig. 1a ). The production of IL-6, TNF-α and RANTES by BM-cDCs was completely inhibited by anti-TLR7 mAb ( Fig. 2b and Supplementary Fig. 2b ). Loxoribine and polyuridylic acid (polyU) induced IFN-α, IL-12 p40 and IL-6 production in BM-pDCs. These responses were significantly inhibited by the anti-TLR7 mAb ( Fig. 2c and Supplementary Fig. 2c ). TLR9 responses in BM-cDCs and BM-pDCs were not altered by the anti-TLR7 mAb ( Fig. 2b and Supplementary Fig. 2c ). Furthermore, B-cell proliferation in response to another TLR7 ligand, imiquimod, was profoundly inhibited ( Fig. 2d ). B-cell proliferation by the TLR9 ligand CpG-B or by anti-IgM was not altered. Next, the effect of the anti-TLR7 mAb on in vivo TLR7 responses was studied. The TLR7 ligand R848 induced IL-6 and IL-12 p40 production in vivo . The mice were administered the anti-TLR7 mAb and, then, 8 h later, R848 and serum IL-6 and IL-12 p40 levels were evaluated 2 h after R848 injection. Cytokine production induced by R848 was significantly downregulated by the anti-TLR7 mAb ( Fig. 2e ). These results demonstrate that the anti-TLR7 mAb specifically inhibits TLR7 responses by a variety of TLR7 ligands in a variety of immune cells in vitro and in vivo . 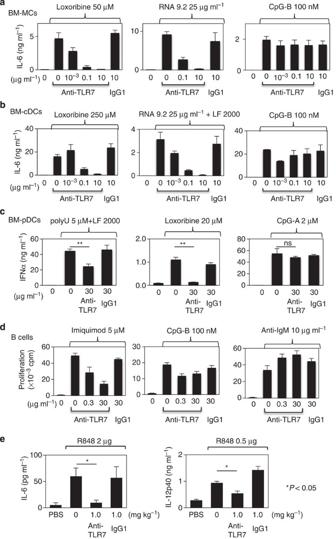Figure 2: Anti-TLR7 mAb inhibits TLR7 responsesin vitroandin vivo. BM-MCs (a), BM-cDCs (b), BM-pDCs (c) and B cells (d) were stimulated with TLR ligands. TLR7 ligands include small chemicals (loxoribine and imiquimod) and oligoRNA (RNA9.2 and polyU). TLR9 ligands include CpG-A and CpG-B. Anti-IgM was also utilized for B-cell activation. Anti-TLR7 mAb (anti-TLR7) or isotype-matched control mAb (IgG1) was added at the indicated concentrations. Cytokine production and B-cell proliferation were evaluated. The results are represented by the mean plus s.d. from triplicate wells. These data are representative of three independent experiments. Statistical analyses were calculated with Student’st-test (**P<0.005, ns: not significant). (e) Mice were intravenously administered anti-TLR7 or IgG1 mAb (4 mg kg−1) 8 h before TLR7 ligand R848 (0.1 mg kg−1for IL-6 and 0.025 mg kg−1for IL-12 p40) stimulation. Blood was collected 2 h after R848 injection, and serum IL-6 and IL-12 p40 levels were measured by ELISA. The results are represented by the mean plus s.d. from four mice. These data are representative of three independent experiments. Statistical analyses were calculated with Student’st-test (*P<0.05). Figure 2: Anti-TLR7 mAb inhibits TLR7 responses in vitro and in vivo. BM-MCs ( a ), BM-cDCs ( b ), BM-pDCs ( c ) and B cells ( d ) were stimulated with TLR ligands. TLR7 ligands include small chemicals (loxoribine and imiquimod) and oligoRNA (RNA9.2 and polyU). TLR9 ligands include CpG-A and CpG-B. Anti-IgM was also utilized for B-cell activation. Anti-TLR7 mAb (anti-TLR7) or isotype-matched control mAb (IgG1) was added at the indicated concentrations. Cytokine production and B-cell proliferation were evaluated. The results are represented by the mean plus s.d. from triplicate wells. These data are representative of three independent experiments. Statistical analyses were calculated with Student’s t -test (** P <0.005, ns: not significant). ( e ) Mice were intravenously administered anti-TLR7 or IgG1 mAb (4 mg kg −1 ) 8 h before TLR7 ligand R848 (0.1 mg kg −1 for IL-6 and 0.025 mg kg −1 for IL-12 p40) stimulation. Blood was collected 2 h after R848 injection, and serum IL-6 and IL-12 p40 levels were measured by ELISA. The results are represented by the mean plus s.d. from four mice. These data are representative of three independent experiments. Statistical analyses were calculated with Student’s t -test (* P <0.05). Full size image Accumulation of the TLR7 immune complex in endolysosomes To address the underlying mechanisms of the inhibitory effect of the anti-TLR7 mAb, the origin of cell surface TLR7 was first studied. The TLR7 ectodomain is proteolytically cleaved in endolysosomes but not in the ER [8] , [20] . Cell surface TLR7 that is proteolytically cleaved is derived from endolysosomes rather than from the ER. BM-MCs were subjected to cell surface biotinylation, immunoprecipitation with anti-TLR7 mAb and immunoprobing with streptavidin. Both full-length TLR7 (TLR7F) and TLR7N were detected by streptavidin from wild-type BM-MCs but not from Tlr7 −/− BM-MCs ( Fig. 3a , lanes 4 and 6). TLR7C was difficult to detect because of the nonspecific signal. Cell surface-specific biotinylation was validated using Unc93b1 3d/3d mice; cell surface TLR7 was not detected on Unc93b1 3d/3d cells ( Fig. 1b ). Consistent with the lack of cell surface TLR7, TLR7F was detected by the anti-TLR7 mAb but not by streptavidin in Unc93b1 3d/3d cells ( Fig. 3a , lanes 2 and 5). Cell surface biotinylation was conducted at room temperature. It is possible that uncleaved TLR7 is internalized during biotinylation and cleaved in endolysosomes. Cell surface biotinylation was also conducted at 4 °C, and cleaved TLR7N was still detectable ( Supplementary Fig. 3 ). These results demonstrate that some of the cell surface TLR7 are cleaved. Cleaved TLR7 on the cell surface is likely to traffic from endolysosomes. 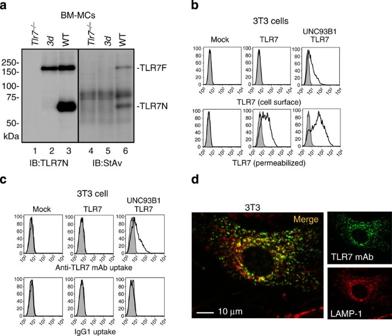Figure 3: The anti-TLR7 mAb–TLR7 immune complex accumulates in endolysosomes. (a) BM-MCs fromTlr7−/−,3dor WT mice were subjected to cell surface biotinylation, immunoprecipitation with the anti-TLR7 mAb and immunoprobing with anti-TLR7N or streptavidin. TLR7F; full-length TLR7; TLR7N, N-terminal cleaved fragment of TLR7. (b) 3T3 fibroblasts expressing TLR7 and/or UNC93B1 were subjected to cell surface or membrane-permeabilized staining using the anti-TLR7 mAb. Grey histograms show staining with the secondary reagent alone. (c) 3T3 fibroblasts expressing TLR7 and/or UNC93B1 were incubated with Alexa Fluor 488-labelled IgG1 or anti-TLR7 mAb for 24 h at 37 °C and were analysed by FACS. (d) 3T3 fibroblasts expressing TLR7, UNC93B1 and LAMP-1-mCherry were incubated with Alexa Fluor 488-labelled anti-TLR7 mAb for 24 h at 37 °C. The fluorescence of the cell surface mAb was quenched, and the distribution of internalized anti-TLR7 mAb was analysed by confocal microscopy. Scale bar, 10 μm. Figure 3: The anti-TLR7 mAb–TLR7 immune complex accumulates in endolysosomes. ( a ) BM-MCs from Tlr7 −/− , 3d or WT mice were subjected to cell surface biotinylation, immunoprecipitation with the anti-TLR7 mAb and immunoprobing with anti-TLR7N or streptavidin. TLR7F; full-length TLR7; TLR7N, N-terminal cleaved fragment of TLR7. ( b ) 3T3 fibroblasts expressing TLR7 and/or UNC93B1 were subjected to cell surface or membrane-permeabilized staining using the anti-TLR7 mAb. Grey histograms show staining with the secondary reagent alone. ( c ) 3T3 fibroblasts expressing TLR7 and/or UNC93B1 were incubated with Alexa Fluor 488-labelled IgG1 or anti-TLR7 mAb for 24 h at 37 °C and were analysed by FACS. ( d ) 3T3 fibroblasts expressing TLR7, UNC93B1 and LAMP-1-mCherry were incubated with Alexa Fluor 488-labelled anti-TLR7 mAb for 24 h at 37 °C. The fluorescence of the cell surface mAb was quenched, and the distribution of internalized anti-TLR7 mAb was analysed by confocal microscopy. Scale bar, 10 μm. Full size image To further study cell surface TLR7, TLR7 with or without Unc93B1 was expressed in 3T3 fibroblasts. Cell surface TLR7 was detected only when Unc93B1 was co-expressed ( Fig. 3b ). 3T3 fibroblasts were incubated with Alexa Fluor 488-labelled TLR7 mAb for 24 h at 37 °C. Fluorescence-activated cell sorting (FACS) analyses revealed that the anti-TLR7 mAb specifically bound to cell surface TLR7-positive 3T3 cells ( Fig. 3c ). Confocal microscopy analysis showed that the anti-TLR7 mAb was internalized into LAMP-1-positive lysosomes ( Fig. 3d ). These results demonstrate that the anti-TLR7 mAb is internalized in a cell surface TLR7-dependent manner. BM-cDCs were studied next. Most of the TLR7 in BM-cDCs was located in the intracellular compartment ( Fig. 1a ). Despite the low expression of cell surface TLR7, the anti-TLR7 mAb at 0.1 and 1 μg ml −1 was internalized into WT BM-cDCs more than in Tlr7 −/− BM-cDCs ( Fig. 4a ). At 1 and 10 μg ml −1 , the anti-TLR7 mAb was internalized into Tlr7 −/− BM-cDCs, suggesting that nonspecific FcR-mediated uptake occurs at higher concentrations. Consistent with this, irrelevant IgG1 at 1 and 10 μg ml −1 was also incorporated into BM-cDCs. The internalization of anti-TLR7 mAb and IgG1 was confirmed by confocal microscopy ( Supplementary Fig. 4 ). FcγRs are expressed on macrophages and DCs but not on 3T3 cells ( Supplementary Fig. 5 ). To address a role of Fc receptors in anti-TLR7 mAb uptake and its inhibitory effect, we studied Fc receptor common γ-chain-deficient ( Fcer1g −/− ) mice. In the absence of FcRγ, IgG internalization into BM-cDCs was apparently decreased ( Fig. 4a ). Despite the impaired IgG1 uptake in Fcer1g −/− BM-cDCs, the inhibitory effect of anti-TLR7 mAb was not altered ( Fig. 4b ), demonstrating that the contribution of FcR-dependent IgG1 internalization on the inhibitory effect of anti-TLR7 mAb is marginal. 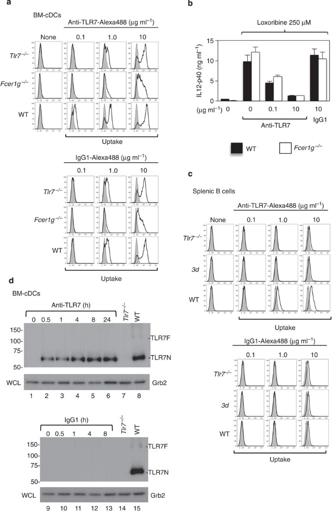Figure 4: The essential role of cell surface TLR7 in the internalization of the anti-TLR7 mAb into BM-cDCs. (a) WT,Fcer1g−/−orTlr7−/−BM-cDCs were incubated with Alexa Fluor 488-labelled anti-TLR7 mAb or IgG1 at the indicated concentration for 24 h at 37 °C. The fluorescence of the cell surface mAb was quenched, and internalized mAbs were analysed by FACS. (b) BM-cDCs from WT andFcer1g−/−mice were pre-treated with anti-TLR7 mAb or IgG1 for 4 h and stimulated with the TLR7 ligand loxoribine. Cytokine production was detected using ELISA. The results are represented by the mean plus SD from triplicate wells. These data are representative of two independent experiments. (c) Uptake of the anti-TLR7 mAb or IgG1 by WT,3d,Tlr7−/−B cells were analysed as described ina. (d) BM-cDCs were incubated with IgG1 or anti-TLR7 mAb for the indicated periods of time. Internalized Abs were precipitated by protein G beads, and TLR7 was immunoprobed. The total amount of TLR7 in BM-cDCs is shown by immunoprecipitation with anti-TLR7 mAb-coupled beads (lanes 8 and 15). TLR7F; full-length TLR7; TLR7N, N-terminal cleaved fragment of TLR7. Lanes 7 and 14 represent the negative controls for TLR7 immunoprecipitation usingTlr7−/−BM-cDCs. Grb2 is shown as a loading control. These data are representative of three independent experiments. Figure 4: The essential role of cell surface TLR7 in the internalization of the anti-TLR7 mAb into BM-cDCs. ( a ) WT, Fcer1g −/− or Tlr7 −/− BM-cDCs were incubated with Alexa Fluor 488-labelled anti-TLR7 mAb or IgG1 at the indicated concentration for 24 h at 37 °C. The fluorescence of the cell surface mAb was quenched, and internalized mAbs were analysed by FACS. ( b ) BM-cDCs from WT and Fcer1g −/− mice were pre-treated with anti-TLR7 mAb or IgG1 for 4 h and stimulated with the TLR7 ligand loxoribine. Cytokine production was detected using ELISA. The results are represented by the mean plus SD from triplicate wells. These data are representative of two independent experiments. ( c ) Uptake of the anti-TLR7 mAb or IgG1 by WT, 3d , Tlr7 −/− B cells were analysed as described in a . ( d ) BM-cDCs were incubated with IgG1 or anti-TLR7 mAb for the indicated periods of time. Internalized Abs were precipitated by protein G beads, and TLR7 was immunoprobed. The total amount of TLR7 in BM-cDCs is shown by immunoprecipitation with anti-TLR7 mAb-coupled beads (lanes 8 and 15). TLR7F; full-length TLR7; TLR7N, N-terminal cleaved fragment of TLR7. Lanes 7 and 14 represent the negative controls for TLR7 immunoprecipitation using Tlr7 −/− BM-cDCs. Grb2 is shown as a loading control. These data are representative of three independent experiments. Full size image To further confirm the TLR7-dependent internalization of anti-TLR7 mAb, we studied B cells, for which FcR is not involved in internalization. Irrelevant IgG1 was hardly internalized into B cells ( Fig. 4c ). In contrast, the anti-TLR7 mAb was internalized into wild-type B cells but not into Tlr7 −/− or Unc93b1 3d/3d B cells, demonstrating that the internalization into B cells is dependent on cell surface TLR7. Despite the lack of FcR-mediated internalization of IgG1, the anti-TLR7 mAb was able to inhibit TLR7 responses in B cells ( Fig. 2d ). Taken together, internalization of the anti-TLR7 mAb with TLR7 is important for its inhibitory effect. To assess the fate of the internalized immune complex, immunoprecipitation of the internalized mAb with protein G beads was conducted. TLR7 was precipitated with internalized anti-TLR7 mAb but not with irrelevant IgG1. The amount of precipitated TLR7 slowly increased, reaching the maximal level at 8 h after mAb addition ( Fig. 4d , lane 5). When compared with total TLR7 (lane 8), most of the TLR7 was precipitated with the anti-TLR7 mAb (compare lanes 6 and 8), demonstrating that most of the TLR7 forms immune complexes with anti-TLR7 mAb. TLR7 in BM-cDCs was mostly cleaved and localized in endolysosomes ( Fig. 4d , lane 8). Nonetheless, exogenously added mAb was able to interact with TLR7. Epitope mapping of the anti-TLR7 mAb The anti-TLR7 mAb was shown to react with the TLR7N fragment from 27 to 457 (ref. 20 ). Taking advantage of the fact that the anti-TLR7 mAb reacts with mouse but not human TLR7, mouse–human TLR7 chimeric molecules were stained with the anti-TLR7 mAb for epitope mapping. The region 275–313 was required for mAb binding ( Fig. 5 ). Recently, the structure of human TLR8 with its ligand was solved, and the ligand-binding domains and dimerization interfaces were identified [23] . The anti-TLR7 mAb epitope is close to the TLR7 regions corresponding to the two ligand-binding sites and one dimerization interface of TLR8: 263Y and 351–356 for ligand-binding and 264–268 for dimerization. These results suggest that the anti-TLR7 mAb disrupts the interaction between TLR7 and its ligands. To address this possibility, a pull-down assay using the TLR7 ectodomain was conducted. Purified TLR7 ectodomain was precipitated by the biotinylated TLR7 ligand CL264 followed by streptavidin. The TLR7 ectodomain was proteolytically cleaved during preparation, and the N-terminal TLR7 fragment (TLR7N) was detected by immunoblotting. The TLR7 ectodomain was precipitated by CL264, but the anti-TLR7 mAb failed to inhibit this precipitation ( Supplementary Fig. 6 ). The anti-TLR7 mAb might disrupt TLR7 dimerization instead of inhibiting the interaction between TLR7 and its ligand. 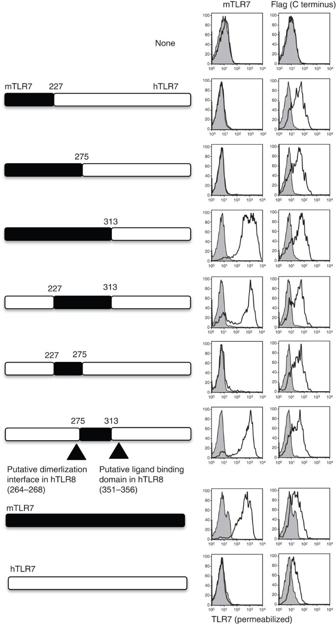Figure 5: Epitope mapping of the TLR7 mAb. Ba/F3 cells expressing flag-tagged mouse TLR7, human TLR7 or mouse/human chimeric TLR7 were subjected to membrane-permeabilized staining with anti-TLR7 mAb or anti-flag. These data are representative of two independent experiments. Figure 5: Epitope mapping of the TLR7 mAb. Ba/F3 cells expressing flag-tagged mouse TLR7, human TLR7 or mouse/human chimeric TLR7 were subjected to membrane-permeabilized staining with anti-TLR7 mAb or anti-flag. These data are representative of two independent experiments. Full size image The efficacy of anti-TLR7 mAb in spontaneous inflammation Finally, the therapeutic effect of anti-TLR7 mAb was studied. The therapeutic effect of the mAb was evaluated in chronic progressive inflammation driven by spontaneous TLR7 activation rather than transient inflammation induced by synthetic TLR7 ligands. Unc93b1 D34A/D34A mice harbouring the D34A mutation suffer from systemic lethal inflammation due to TLR7 hyper-responsiveness [14] . Systemic inflammation causes thrombocytopenia, splenomegaly and chronic active hepatitis. Given that Unc93B1 controls TLR7 distribution, it is important to study the effect of the D34A mutation of the Unc93B1 gene on TLR7 cell surface expression. Membrane-permeabilized staining revealed that the total amount of TLR7 was not altered in Unc93b1 D34A/D34A immune cells, including B cells, macrophages and DCs ( Fig. 6 and Supplementary Fig. 7 ). Although B cells have been shown to be pathogenic in Unc93b1 D34A/D34A mice [14] , no apparent increase in cell surface TLR7 expression was observed in Unc93b1 D34A/D34A B cells ( Fig. 6a ). Notably, cell surface TLR7 on Unc93b1 D34A/D34A BM-MCs was apparently lower than wild-type BM-MCs ( Fig. 6b ). Furthermore, an increase in cell surface TLR7 expression was not observed in other types of cells, including neutrophils, inflammatory monocytes and DC subsets ( Fig. 6b and Supplementary Fig. 7 ). 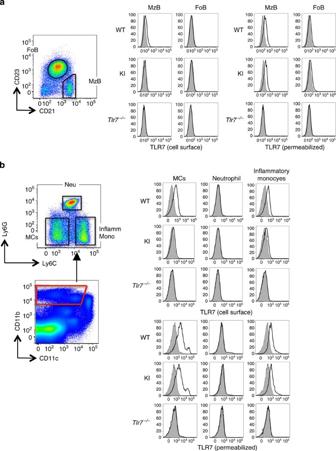Figure 6: Cell surface expression of TLR7 inUnc93b1D34A/D34Amice. (a) The dot plot shows the cell surface expression of CD21 and CD23 on CD19-positive splenic B cells. The gates indicate marginal zone (Mz) and follicular (Fo) B cells. Histograms show the cell surface (left) and total (right) TLR7 on Mz and Fo B cells from WT,Unc93b1D34A/D34A(KI) orTlr7−/−mice. Grey histograms show staining with the secondary reagent alone. (b) The lower dot plot shows CD11c and CD11b expression on splenic cells. The upper dot plot shows cell surface Ly6G and Ly6C expression on the cell population gated in the lower dot plot. The gates indicate macrophages (MC), monocytes and neutrophils. Open histograms show cell surface (top) and total TLR7 (bottom) expression in macrophages, neutrophils and inflammatory monocytes. These data are representative of two independent experiments. Figure 6: Cell surface expression of TLR7 in Unc93b1 D34A/D34A mice. ( a ) The dot plot shows the cell surface expression of CD21 and CD23 on CD19-positive splenic B cells. The gates indicate marginal zone (Mz) and follicular (Fo) B cells. Histograms show the cell surface (left) and total (right) TLR7 on Mz and Fo B cells from WT, Unc93b1 D34A/D34A (KI) or Tlr7 −/− mice. Grey histograms show staining with the secondary reagent alone. ( b ) The lower dot plot shows CD11c and CD11b expression on splenic cells. The upper dot plot shows cell surface Ly6G and Ly6C expression on the cell population gated in the lower dot plot. The gates indicate macrophages (MC), monocytes and neutrophils. Open histograms show cell surface (top) and total TLR7 (bottom) expression in macrophages, neutrophils and inflammatory monocytes. These data are representative of two independent experiments. Full size image The anti-TLR7 mAb was injected every week into Unc93b1 D34A/D34A mice that had already suffered from thrombocytopenia. Two out of ten mice died during treatment with control IgG1, whereas none out of eleven mice died during treatment with the anti-TLR7 mAb. After 10 weeks, the platelet counts in mice treated with the anti-TLR7 mAb were significantly recovered ( Fig. 7a ). After mAb treatment, the mice were killed for the analyses of splenomegaly and hepatitis. Splenomegaly in mice treated with the anti-TLR7 mAb was significantly milder than those treated with IgG1 ( Fig. 7b ). The serum titre of anti-Sm Ab, an RNA-specific autoAb, was measured. The mice treated with the anti-TLR7 mAb showed significantly lower anti-Sm Ab titres than the mice treated with control IgG1 ( Fig. 7c ). Finally, hepatitis was assessed by histological analyses using the Knodell HAI score ( Fig. 7d ) [24] . Mononuclear cell infiltration in portal/periportal and intralobular areas, piecemeal necrosis with destruction of individual hepatocytes along the edges of the portal tract ( Fig. 7e,f , black arrowhead), focal hepatocellular necrosis ( Fig. 7f , white arrowhead) and fibrosis ( Fig. 7h ) indicated chronic active hepatitis in Unc93b1 D34A/D34A mice. These indicators of hepatitis were not apparent in mice treated with the anti-TLR7 mAb ( Fig. 7g,i ). These results demonstrate the therapeutic effect of the anti-TLR7 mAb on TLR7-dependent systemic inflammation. 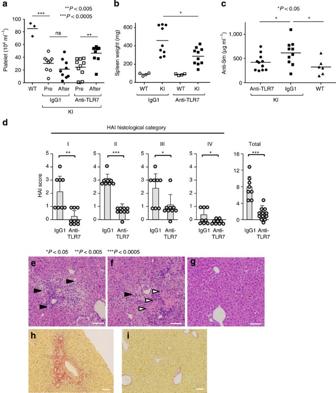Figure 7: Anti-TLR7 mAb ameliorates inflammation caused by Unc93b1 mutation. (a–c) WT andUnc93b1D34A/D34A(KI) mice ~4-month old were intravenously injected with 4 mg kg−1IgG1 (n=8) or anti-TLR7 mAb (n=9) every week for 10 weeks. Platelet counts (a), spleen weights (b) and anti-Sm Ab titres (c) of WT and KI mice before and after mAb treatment are shown. (d) The Knodell HAI score for the livers in KI mice treated with IgG1 or with anti-TLR7 mAb is shown. The HAI score is graded in four categories: I, periportal and/or bridging necrosis; II, intralobular degeneration and focal hepatocellular necrosis; III, portal inflammation; and IV, fibrosis.Circlesindicate each individual,Barsindicate the average of each group and theerror barsindicate the s.d. (e–g) Histological staining with haematoxylin and eosine (H&E) of KI mouse livers treated with IgG1 (e,f) or with anti-TLR7 mAb (g). KI mice treated with IgG1 show a prominent mononuclear cell infiltration in the portal/periportal and intralobular areas, piecemeal necrosis with destruction of individual hepatocytes along the edges of the portal tract (black arrowhead) and focal hepatocellular necrosis (white arrowhead). Scale bars, 100 μm. (h,i) Picrosirius red staining was performed to detect fibrosis in the livers of KI mice treated with IgG1 (h) or anti-TLR7 mAb (i). Statistical analyses were calculated with Student’st-test (*P<0.05, **P<0.005, ***P<0.0005, ns: not significant). Figure 7: Anti-TLR7 mAb ameliorates inflammation caused by Unc93b1 mutation. ( a – c ) WT and Unc93b1 D34A/D34A (KI) mice ~4-month old were intravenously injected with 4 mg kg −1 IgG1 ( n =8) or anti-TLR7 mAb ( n =9) every week for 10 weeks. Platelet counts ( a ), spleen weights ( b ) and anti-Sm Ab titres ( c ) of WT and KI mice before and after mAb treatment are shown. ( d ) The Knodell HAI score for the livers in KI mice treated with IgG1 or with anti-TLR7 mAb is shown. The HAI score is graded in four categories: I, periportal and/or bridging necrosis; II, intralobular degeneration and focal hepatocellular necrosis; III, portal inflammation; and IV, fibrosis. Circles indicate each individual, Bars indicate the average of each group and the error bars indicate the s.d. ( e – g ) Histological staining with haematoxylin and eosine (H&E) of KI mouse livers treated with IgG1 ( e , f ) or with anti-TLR7 mAb ( g ). KI mice treated with IgG1 show a prominent mononuclear cell infiltration in the portal/periportal and intralobular areas, piecemeal necrosis with destruction of individual hepatocytes along the edges of the portal tract (black arrowhead) and focal hepatocellular necrosis (white arrowhead). Scale bars, 100 μm. ( h , i ) Picrosirius red staining was performed to detect fibrosis in the livers of KI mice treated with IgG1 ( h ) or anti-TLR7 mAb ( i ). Statistical analyses were calculated with Student’s t -test (* P <0.05, ** P <0.005, *** P <0.0005, ns: not significant). Full size image The present study shows that TLR7 can be targeted by Ab-mediated intervention. Use of the anti-TLR7 mAb clearly demonstrated that TLR7 is expressed on the surface of macrophages and DCs in the spleen. Both cleaved and uncleaved TLR7 are expressed on the cell surface. Cleaved TLR7 likely traffics from the endolysosomes, whereas uncleaved TLR7 is from the ER. TLR7 trafficking from the ER to the cell surface correlates with TLR7 protein synthesis. However, TLR7 trafficking from the endolysosomes to the cell surface likely results from lysosomal exocytosis. Lysosomes specialized for secretion are known as lysosome-related organelles (LROs), where TLR7 and TLR9 are localized and deliver a signal [25] , [26] . AP-3 and the Hermansky–Pudlak syndrome proteins BLOC-1 and BLOC-2 have been shown to play a role in LRO biogenesis and TLR7/9 responses [25] , [26] . Cell surface TLR7 is likely tightly linked with LRO trafficking and function. Cell surface expression of TLR9 has been recently reported [21] , [27] . One anti-TLR9 mAb detects TLR9 in membrane-permeabilized staining but not in cell surface staining [21] . In contrast, the other anti-TLR9 mAb is able to detect TLR9 in both membrane-permeabilized and cell surface staining. These results suggest that cell surface TLR9 is distinct from endolysosomal TLR9 in its conformation. Proteolytic processing does not explain this difference because both mAbs are able to detect both cleaved and uncleaved TLR9. Considering that the enforced expression of TLR9 on the cell surface leads to systemic lethal inflammation [11] , cell surface TLR9 in the steady-state might be silenced. The unique conformation of cell surface TLR9 might reflect a functional difference from endosomal TLR9. Surprisingly, human and mouse neutrophils express functional cell surface TLR9, which induces neutrophil activation [27] . Functional cell surface TLR9 is likely restricted to neutrophils [11] . The present study failed to detect cell surface TLR7 on splenic neutrophils. It is still possible, however, that cell surface TLR7 is induced upon neutrophil activation. A role of cell surface TLR7 in RNA-sensing needs to be addressed in future studies. Unc93B1 is required for the trafficking of TLR7 and TLR9 to the cell surface [21] . Unc93B1 plays a role in TLR trafficking not only to endolysosomes but also to the plasma membrane. Furthermore, an indispensable role of Unc93B1 in the cell surface expression of TLR5 has been recently shown [28] . TLR5 is a cell surface TLR that shows a distinct distribution from TLR7 and TLR9. Unc93B1 controls a variety of TLR-trafficking pathways. It is important to understand how one single molecule controls the distinct trafficking pathways of several TLRs. Although only a small amount of TLR7 was detected on the surface of BM-cDCs, most of the TLR7 in endolysosomes were detected as immune complexes. Considering that cell surface TLR7 was partially cleaved, cleaved TLR7 is likely to come from endolysosomes, suggesting that TLR7 is trafficked from the endolysosomes to the cell surface. Our results indicate that cell surface TLR7 forms immune complexes with the anti-TLR7 mAb and internalizes into endolysosomes. If TLR7 trafficking from endolysosomes to the cell surface continuously occurs or is induced by the anti-TLR7 mAb, the anti-TLR7 mAb would be able to interact with most of the TLR7, despite the very low TLR7 expression on the cell surface. This possibility needs to be addressed in future studies. Although IgG1 internalization was impaired in Fcer1g −/− BM-cDCs, the inhibitory effect of the anti-TLR7 mAb was not altered. Moreover, the inhibitory effect of the anti-TLR7 mAb was observed in B cells, in which FcR-mediated IgG1 internalization was negligibly low. Internalization of the anti-TLR7 mAb into B cells was dependent on cell surface TLR7. Although only a small amount of TLR7 was expressed on the surface of B cells and BM-cDCs, the mAb apparently inhibited TLR7 responses that occur in endolysosomes. Internalization of the TLR7 immune complex is likely important for the inhibitory effect of the anti-TLR7 mAb. The immune complexes were stable for as long as 24 h in endolysosomes. The anti-TLR7 mAb bound to the TLR7 ectodomain but failed to interfere with the interaction between the TLR7 ectodomain and its ligand. The anti-TLR7 mAb might inhibit TLR7 responses by interfering with TLR7 dimerization. It is also possible that the anti-TLR7 mAb changes the distribution of TLR7 and thereby negatively regulates TLR7 responses. TLR7 belongs to the group of endolysosomal antigens that includes CD63. CD63 is expressed on the cell surface and in secretory lysosomes [29] . Notably, an anti-CD63 mAb is able to inhibit allergic reactions [30] . It is possible that the CD63 mAb is internalized and thereby inhibits the degranulation of mast cells. Although the major targets of mAb-mediated intervention have been cell surface receptors and secreted cytokines, endolysosomal molecules can also be modulated by mAbs. mAbs are stable and remain active in endolysosomes. The present study has expanded the target list for Ab-mediated intervention to include endolysosomal molecules. Unc93b1 D34A/D34A mice suffer from thrombocytopenia, splenomegaly and hepatitis. These types of systemic inflammation are activated by TLR7 expressed in B cells [14] . Macrophages and DCs might also contribute to the systemic inflammation. The anti-TLR7 mAb inhibited TLR7 responses of B cells, DCs and macrophages in vitro . The inhibitory effect of the anti-TLR7 mAb ameliorated a variety of inflammatory symptoms observed in Unc93b1 D34A/D34A mice. TLR7 has been implicated in a variety of autoimmune diseases [6] , [31] . By using inhibitory oligodeoxynucleotides, TLR7 has been shown to be a promising target for therapeutic intervention in mouse models of psoriasis and SLE [18] , [19] . The present study has revealed that the anti-TLR7 mAb is another powerful tool for therapeutic intervention in a variety of autoimmune diseases. Reagents and Abs CpG-A 1585 (5′- G*G*GGTCAACGTTGAG*G*G*G*G*G -3′, asterisks indicate phosphorothioated residues) and RNA9.2s-DR (5′- UGUCCUUCAAUGUCCUUCAA -3′, all phosphorothioated) [22] , PolyU (5′- UUUUUUUUUUUUUUUUUUU -3′, all phosphorothioated) were synthesized by Hokkaido System Science. CpG-B 1688 (5′- TCCATGACGTTCCTGATGCT -3′, all phosphorothioated) was synthesized by FASMAC. Loxoribine (7-allyl-7,8-dihydro-8-oxo-guanosine) was purchased from Enzo Life Science. Imiquimod (R837) and R848 were purchased from InvivoGen. Digitonin was purchased from Nacalai Tesque. Lipofectamine 2000 reagent was purchased from Invitrogen. Saponin was purchased from Sigma-Aldrich. The anti-TLR7 mAb was previously established by us [20] . The anti-TLR7 mAb was purified from ascitic fluid. Isotype-matched IgG1 mAb was similarly purified and used as a control mAb. Plasmid constructs The flag epitope was tagged to the C termini of mouse TLR7, human TLR7 or their chimeric constructs. The cherry epitope was tagged to the C terminus of mouse Lamp1. The constructs were generated by PCR and cloned into retroviral pMX vectors (kindly provided by Dr T. Kitamura, The University of Tokyo, Japan). Mice C57BL/6 mice were purchased from Japan SLC Inc. (Shizuoka, Japan). Tlr7 −/− and Fcer1g −/− mice were kindly given by Professors S. Akira (Osaka University, Japan) and T. Takai (Tohoku University, Japan), respectively. Unc93B1 3d/3d mice were kindly provided by Professor B. Beutler (The Scripps Research Institute, USA). Un93b1 D34A/D34A mice were generated in our laboratory [14] . These mutant mice were backcrossed to the C57BL/6 strain, and male mice aged 6–12 weeks old were used. Female Un93b1 D34A/D34A mice injected with the mAb were used at 16 weeks old. Mice were maintained in the animal facility of the Institute of Medical Science at the University of Tokyo, and all mouse experiments were approved by the Institutional Animal Care and Use Committee. Cell lines Ba/F3 cells were cultured in Roswell Park Memorial Institute (RPMI) 1640 medium supplied with 10% FBS, IL-3, penicillin–streptomycin–glutamine and 50 μM 2-ME. NIH3T3, RAW264.7, P388D1 and J774 cells were cultured in DMEM supplied with 10% FBS, penicillin–streptomycin–glutamine and 50 μM 2-ME. Retroviral transduction pMX vectors were transfected into Plat-E packaging cells with FuGene6 (Roche). After 2-day incubation, the supernatant was obtained as a viral suspension. Cells were infected by a mixture of the viral suspension and DOTAP (Roche). Induction of BM-DCs and macrophages BM-cDCs and BM-pDCs were induced by culturing with 10 ng ml −1 of murine granulocyte–macrophage colony-stimulating factor (PeproTech) and 100 ng ml −1 of fms -like tyrosine kinase-3 ligand (Flt3L, PeproTech), respectively, in 10% FBS, penicillin–streptomycin–L-glutamine, 50 μM 2-ME-containing RPMI 1640 medium for 7 days. For BM-pDCs, the CD11c + B220 + population was isolated with a FACSAria flow cytometer. BM-MCs were induced by culturing with 10 ng ml −1 of murine M-CSF (PeproTech) in 10% FBS, penicillin–streptomycin–L-glutamine and 50 μM 2-ME-containing DMEM for 7 days [15] . Enzyme-linked immunosorbent assay (ELISA) Cytokine and interferon levels in the culture supernatant were measured with ELISA kits (R&D Systems). IL-6 and IL-12 p40 in mouse serum were measured with ELISA kits (eBioscience). For the ELISA detecting anti-Sm Ab, 50 μg ml −1 Sm antigen (ImmunoVision) was coated on a 96-well half-area plate (Greiner Bio-One), blocked with 3% BSA in PBS and incubated with diluted sera (1:100). After washing with 0.05% Tween 20 in PBS, the samples were reacted with horseradish peroxidase (HRP)-conjugated anti-mouse Ig(H+L) Ab (1:15,000; Southern Biotech). The monoclonal Ab Y12 (Abcam) was used as the standard. B-cell proliferation assay Splenocyte B cells were obtained from 6- to 12-week-old mice and were enriched by negative selection using CD43 magnetic microbeads (Miltenyi Biotec). The enriched B cells contained more than 90% B220-positive cells. B cells were cultured with ligands or anti-mouse IgM (Jackson ImmunoResearch) in 96-well plates at a density of 6.7 × 10 5 cells ml −1 . After 3 days, B cells were labelled with 1 μCi per well of 3 H-thymidine (PerkinElmer) for 5 h and then subjected to the Cell Harvester (Inotech Biosystems). The 3 H-thymidine uptake was measured by Microbeta (PerkinElmer), following the manufacturer’s instructions. Confocal imaging 3T3 cells overexpressing Lamp-1-mCherry and BM-cDCs were incubated with purified anti-TLR7 mAb for 24 h, fixed in 4% paraformaldehyde for 10 min and then permeabilized with 0.1% Triton X-100 in 2.5% BSA containing BlockingOne (Nacalai Tesque) for 30 min. The cells were incubated with anti-mouse IgG Abs conjugated to Alexa Fluor 488 (1:1,000; Invitrogen) for 90 min at 37 °C. These cells were examined under an LSM 710 confocal microscope using a × 63 NA1.4 Plan-Apochromat oil immersion lens (Zeiss). Images were acquired and analysed using the ZEN software (Zeiss). At least three independent experiments were conducted for each image. Flow cytometry Cells were pre-incubated with anti-FcμRII/FcμRIII (1:1,000; 93) for blocking and were stained with fluorescein-conjugated Abs specific to the following markers for flow cytometry analysis: B220-FITC (1:1,000; RA3-6B2), CD8a APC-eFluor780 (1:1,000; 53-6.7), CD11b-FITC (1:800; M1/70), CD11c-PE-Cy7 (1:2,000; N418) and CD11c-APC (1:2,000; N418), all purchased from eBioscience; CD11b-BV510 (1:800; M1/70) and Ly6G-APC (1:2,500; 1A8), purchased from BD Pharmingen; PDCA1-FITC (1:600; 927), Ly6C-FITC (1:1,500; HK1.4), CD19-PE-Cy7 (1:1,000; 6D5), FcμRII/FcμRIII-PE-Cy7 (1:3,000; 93), CD23-APC (1:1,000; B3B4) and CD21-BV421 (1:800; CR2/CR1), purchased from BioLegend. Cells were incubated at 4 °C with biotinylated anti-TLR7 mAbs (1:3,000; A94B10) diluted in staining buffer (1 × PBS with 2.5% FBS and 0.1% NaN 3 ), followed by incubation with streptavidin-PE (1:3,000; eBioscience). For the intracellular staining, cells were permeabilized with 0.1% saponin containing staining buffer, and subsequent steps were performed with saponin buffer. The flag-tagged-TLR7 in Ba/F3 cells was stained with biotinylated anti-flag Ab (M2; 1:3,000; Sigma-Aldrich). Stained cells were analysed by the FACSCalibur, FACSAria or FACS LSRFortessa (BD Biosciences). Immunoprecipitation BM-MCs were washed twice with HBSS and were subjected to cell surface biotinylation with EZ-Link Sulfo-NHS-LC Biotin (Thermo Scientific) for 1 h at room temperature or 1 h on ice. After washing with HBSS, BM-MCs were lysed in 1% digitonin lysis buffer (20 mM Tris/HCl pH 7.4, 150 mM NaCl, 1 mM CaCl 2 , 1 mM MgCl 2 , 10% Glycerol, 1 × Complete EDTA-free cocktail (Roche Applied Science)). Cell lysates were incubated on ice for 30 min and centrifuged to remove the debris and nuclei. Lysates were collected and rotated at 4 °C for 2 h with the monoclonal Abs against TLR7 or streptavidin-conjugated, NHS-activated Sepharose 4 Fast Flow beads (GE Healthcare). After incubation, the beads were washed three times with 0.1% digitonin washing buffer (20 mM Tris/HCl pH 7.4, 150 mM NaCl, 1 mM CaCl 2 , 1 mM MgCl 2 , 10% Glycerol). For the internalized anti-TLR7 mAb in BM-cDCs, cells were washed twice with PBS and lysed with 1% Triton X-100 lysis buffer (20 mM Tris/HCl pH 7.4, 150 mM NaCl, 1 mM CaCl 2 , 1 mM MgCl 2 , 10% Glycerol, 1 × Complete EDTA-free cocktail). Cell lysates were collected and rotated at 4 °C for 2 h with protein G-conjugated Sepharose 4 Fast Flow beads (GE Healthcare). Immunoprecipitates were subjected to SDS–PAGE after being eluted in sample buffer (62.5 mM Tris/HCl pH 6.8, 10% glycerol, 2% SDS, 0.025% bromophenol blue, 5% 2-ME). After electrophoresis, gel samples were transferred to polyvinylidene difluoride membranes and subjected to immunoblotting with either anti-TLR7N pAb (1:2,000; eBioscience) or streptavidin-HRP (1:3,000; GE Healthcare). The images presented in Figs 3a and 4d were cropped at the putative molecular size, and the full images are shown in Supplementary Figs 8 and 9 , respectively. Preparation of purified mouse TLR7 protein The DNA encoding the extracellular domain of mouse TLR7 (aa 27-840) with a C-terminal thrombin cleavage site followed by a protein A tag was inserted into the expression vector pMT/BiP/V5-His of the Drosophila expression system. Drosophila S2 cells were co-transfected with the TLR7 and pCoHygro vectors. Stably transfected cells were selected in Sf-900 II SFM medium containing 300 μg ml −1 hygromycin. Protein secreted to the supernatant was purified by IgG Sepharose 6 Fast Flow (GE healthcare) affinity chromatography, followed by Superdex 200 gel filtration chromatography. To mimic the Z-loop processing, the protein was incubated with 1/200 (w/w) bovine trypsin for 2 h to cleave the Z-loop and protein A tag. After proteolytic processing, the N- and C-terminal halves of TLR7 remained associated. Z-loop-processed TLR7 was further purified by Superdex 200 gel filtration chromatography (GE Healthcare). Pull-down assay TLR7 ectodomain protein (1 μg) was incubated with either anti-TLR7 mAb (100 μg) or control mAb (100 μg) for 1 h on ice and then was subjected to a pull-down assay with biotinylated CL264 (10 μg) and was precipitated with streptavidin or proG Dynabeads (Life Technologies) for 15 min at room temperature. The Dynabeads were washed three times with washing buffer (5 mM Tris-HCl pH 7.5, 0.5 mM EDTA, 150 mM NaCl, 0.1% Tween). After washing, the beads were eluted by boiling in sample buffer (125 mM Tris/HCl pH 6.8, 20% glycerol, 2% SDS, 0.05% bromophenol blue, 5% 2-ME) at 95 °C for 2 min. The samples were subsequently analysed using SDS–PAGE. After electrophoresis, gel samples were transferred to PVDF membranes and subjected to immunoblotting with anti-TLR7N pAb (1:2,000). The images presented in Supplementary Fig. 6 were cropped at the putative molecular size, and the full images are shown in Supplementary Fig. 11 . HAI Score Histological chronic active hepatitis activity was assessed as previously described [24] . Histological activities were analysed and scored, focusing on the lobules with the most marked inflammation in each specimen. Using the Knodell HAI scoring system, liver specimens were graded into three categories (I–III) for necroinflammation and 1 (IV) for fibrosis. Category I, periportal and/or bridging hepatocellular necrosis, was graded from 0 to 10, where 0=none, 1=mild piecemeal necrosis, 3=moderate piecemeal necrosis (involves less than 50% of the circumference of most portal tracts), 4=marked piecemeal necrosis (involves more than 50% of the circumference of most portal tracts), 5=moderate piecemeal necrosis plus bridging necrosis, 6=marked piecemeal necrosis plus bridging necrosis and 10=multilobular necrosis. Category II, intralobular degeneration and focal hepatocellular necrosis, was graded from 0 to 4, where 0=none, 1=mild (acidophilic bodies, ballooning degeneration and/or scattered foci of hepatocellular necrosis in less than one-third of lobules or nodules), 3=moderate (involvement of one-third to two-thirds of lobules or nodules) and 4=marked (involvement of more than two-thirds of lobules or nodules). Category III, portal inflammation, was graded from 0 to 4, where 0=no portal inflammation, 1=mild (sprinkling of inflammatory cells in less than one-third of portal tracts), 3=moderate (increased inflammatory cells in one-third to two-thirds of portal tracts) and 4=marked (dense packing of inflammatory cells in more than two-thirds of portal tracts). Category IV, fibrosis, was graded from 0 to 4, where 0=no fibrosis, 1=fibrous portal expansion, 3=bridging fibrosis (portal–portal or portal–central linkage) and 4=cirrhosis. Statistical analysis Statistical significance was calculated with a two-tailed unpaired Student’s t -test. P <0.05 was considered statistically significant. How to cite this article: Kanno, A. et al . Targeting cell surface TLR7 for therapeutic intervention in autoimmune diseases. Nat. Commun. 6:6119 doi: 10.1038/ncomms7119 (2015).